Genomic insights into multidrug-resistance, mating and virulence inCandida aurisand related emerging species Candida auris is an emergent multidrug-resistant fungal pathogen causing increasing reports of outbreaks. While distantly related to C. albicans and C. glabrata , C. auris is closely related to rarely observed and often multidrug-resistant species from the C. haemulonii clade. Here, we analyze near complete genome assemblies for the four C. auris clades and three related species, and map intra- and inter-species rearrangements across the seven chromosomes. Using RNA-Seq-guided gene predictions, we find that most mating and meiosis genes are conserved and that clades contain either the MTL a or MTL α mating loci. Comparing the genomes of these emerging species to those of other Candida species identifies genes linked to drug resistance and virulence, including expanded families of transporters and lipases, as well as mutations and copy number variants in ERG11 . Gene expression analysis identifies transporters and metabolic regulators specific to C. auris and those conserved with related species which may contribute to differences in drug response in this emerging fungal clade. Candida auris is an emerging fungal pathogen of increasing concern due to high drug resistance and high mortality rates [1] , [2] . In addition, outbreaks have been reported in hospital settings, suggesting healthcare transmission [2] , [3] . C. auris clinical isolates are typically multidrug-resistant (MDR), with common resistance to fluconazole and variable susceptibility to other azoles, amphotericin B, and echinocandins [2] . C. auris causes bloodstream and other invasive and superficial infections, similar to a group of rarely observed, phylogenetically related species including Candida haemulonii , Candida duobushaemulonii , and Candida pseudohaemulonii [4] , [5] . These species also display MDR, most commonly to amphotericin B and also reduced susceptibility to azoles and echinocandins [4] , [5] . Together, C. auris and these closely related species represent an emerging clade of invasive fungal pathogens, which are not only difficult to treat, but also difficult to identify using standard laboratory methods [6] , generally requiring molecular methods for proper identification. Initial whole genome analysis of C. auris isolates from Pakistan, India, South Africa, Japan, and Venezuela identified four clades that are specific to each geographic region, suggesting that each of these clades emerged nearly simultaneously in different regions of the world [2] . Including data from other recent studies, the current representation of each clade is as follows: clade I comprises isolates from India, Pakistan, and the UK [2] , [3] , [7] , clade II from Japan and South Korea [2] , [8] , clade III from South Africa, and clade IV from Venezuela [2] . Analyses of SNPs identified from whole genome sequence [2] , [9] and of multilocus sequence typing (MLST) [10] , [11] found low genetic diversity between isolates within each C. auris clade. Little is known about whether phenotypic differences exist among isolates from different C. auris clades; one noted difference is that isolates from India and South Africa are capable of assimilating N-acetylglucosamine while isolates from Japan and South Korea were not able to process this compound [2] . Phylogenetic studies revealed that C. auris belongs to the C. haemulonii clade and is distantly related to the more common human pathogenic species including Candida albicans and Candida glabrata [4] , [5] , [12] , [13] . However, these prior studies have not clearly resolved the relationships of species within the C. haemulonii clade, including C. haemulonii, C. duobushaemulonii , and C. pseudohaemulonii [4] , [5] , [12] , [13] . Candida lusitaniae , a rarely observed cause of infection [14] , is a sister clade to this group of emerging species [13] , [15] . Despite the fact that C. auris is highly divergent from other Saccharomycetales yeasts from the CTG clade, which includes the common human pathogens C. albicans , Candida tropicalis , and Candida parapsilosis , most of our limited current knowledge of C. auris resistance and virulence had been inferred based on conservation of genes associated with drug resistance and virulence in C. albicans or in C. glabrata , which is part of the distantly related Nakaseomyces clade. Initial comparative analysis of the gene content of one isolate of C. auris with C. albicans found that some orthologs associated with antifungal resistance are present in C. auris , including drug transporters, secreted proteases, and manosyl transferases [13] . In addition, preliminary genomic studies showed that the targets of several classes of antifungal drugs are conserved in C. auris , including the azole target lanosterol 14 α-demethylase ( ERG11 ), the echinocandin target 1,3-beta-glucan synthase ( FKS1 ), and the flucytosine target uracil phosphoribosyl-transferase ( FUR1 ) [2] , [16] . Furthermore, point mutations associated with drug resistance in other species are observed in many clinical isolates and are associated with C. auris clades [2] , [7] , [16] . Recently, two ERG11 mutations (Y132F and K143R) in C. auris were found to increase resistance to fluconazole [17] , however the role of other genes in drug resistance and virulence has not been reported for this group of emerging MDR species. While efforts to sequence C. auris genome provided an initial view of genome content [9] , [13] , available assemblies in GenBank are highly fragmented, inconsistently annotated, and do not provide a complete representation of all C. auris clades. The related species C. haemulonii and C. duobushaemulonii were recently sequenced [18] , [19] . Here, we generate and annotate highly complete genome assemblies for isolates from each of the clades of C. auris as well as for the related species C. haemulonii , C. duobushaemulonii , and C. pseudohaemulonii . Comparison of these genomes to other sequenced Candida species reveals that C. auris has notable expansions of genes linked to drug resistance and virulence in C. albicans , including families of oligopeptide transporters, siderophore-based iron transporters, and secreted lipases. Using RNA-Seq we examine the response of two isolates of C. auris to antifungal drugs and detect the upregulation of transporters and metabolic regulators that have been previously associated with drug resistance in C. albicans . In addition, we also observe that several either unique or expanded genes in C. auris and related species are upregulated in response to azole and amphotericin B exposure. We also find evidence that C. auris may be capable of mating and meiosis, based on the identification of both mating types in the populations, conservation of genes involved in mating and meiosis, and detection of chromosomal rearrangements between two clades. These results reveal fundamental insights into the evolution of drug resistance and pathogenesis in C. auris and closely related species and the potential for mating and recombination between the C. auris clades. Genome features of Candida auris and closely related species We generated highly complete genome assemblies for four C. auris isolates and for three phylogenetically related species, C. haemulonii , C. duobushaemulonii , and C. pseudohaemulonii . 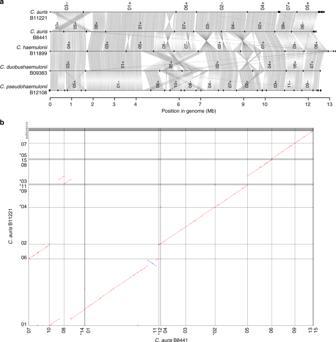Fig. 1 Whole genome conservation, structure, and synteny.aGenome wide gene synteny amongCandida auris,C. haemulonii,C. duobushaemulonii, andC. pseudohaemulonii. To determine synteny regions of conserved gene order, we identified orthologs between these isolates and then plotted chains of orthologs (gray lines). Isolate names are shown to the left of their genomes, which are represented by horizontal black lines, with vertical lines indicating scaffold borders, and their identifiers listed above (+/− = orientation).bShared synteny regions based on whole genome alignments betweenC. aurisB8441 and B11221. Asterisk refers to scaffolds in reverse orientation Most of these isolates displayed increased resistance to fluconazole and also increased resistance to voriconazole or amphotericin B (Supplementary Table 1 ). The C. auris assemblies represent each of the four major clades [2] , including an updated assembly for strain B8441 (clade I) and the first representatives of clade II (strain B11220), clade III (strain B11221), and clade IV (strain B11243). As C. auris is distantly related to other previously sequenced Candida species, we also sequenced genomes of the closely related species C. haemulonii (strain B11899), C. duobushaemulonii (strain B09383), and C. pseudohaemulonii (strain B12108) to enable comparative genomic analysis. The genome assemblies of C. auris (B8441 and B11221), C. haemulonii , and C. duobushaemulonii were sequenced using PacBio and Illumina, whereas the other two C. auris strains and C. pseudohaemulonii were sequenced only with Illumina (Table 1 ; Methods). The genome assemblies of C. auris range from 12.1 Mb in B11220 to 12.7 Mb in B11221. The C. auris B8441 and B11221 genome assemblies were organized in 15 and 20 scaffolds, respectively, of which 7 scaffolds included most of the sequenced bases in both strains (Table 1 ). This represents an improvement upon the previously generated genome assembly of C. auris strain 6684 (clade I) [13] , which consists of 99 scaffolds (759 contigs) that include contig gaps and has an inflated number of predicted genes, based on our analysis (see below; Methods). The genome assemblies of Illumina data for C. auris B11220 (clade II) and B11243 (clade IV) are less contiguous than the assemblies that included long reads, consisting of 324 or 285 contigs, respectively (Table 1 ). The genome assemblies of C. haemulonii , C. duobushaemulonii , and C. pseudohaemulonii were also highly contiguous with 11, 7, and 36 scaffolds, respectively (Table 1 ). 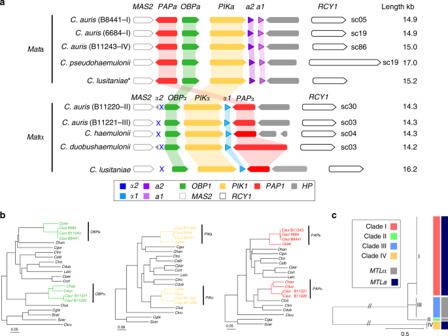Fig. 2 Mating-type loci (MTL) inCandida aurisand closely related species.aSynteny schema depicting the orientation and conservation of the color-codedMTLidiomorphs and genes adjacent to theMTL. The putative MTL inC. auris,C. haemulonii,C. duobushaemulonii, andC. pseudohaemuloniiare shown in comparison with theMTLaandMTLα idiomorphs fromC. lusitaniae.bPhylogenetic analysis of the non-mating flanking genes (PIK1/OBP1/PAP1) showing the inheritance of idiomorphs of these genes within theMTLaandMTLα loci. Branch lengths indicate the mean number of changes per site.cPhylogenetic tree ofC. aurisisolates from Lockhart et al.2. Isolates are color-coded according to the clades (I, II, III, and IV) and mating type (MTLaandMTLα). Supplementary Figure3shows isolates, origin, and the normalized depth read coverage of mapped positions for all isolates aligned to B8441 (MTLa) and B11221 (MTLα), supporting the classification intoMTLaorMTLα Comparison of these four C. auris genomes and those of the three related species revealed that the genome sizes are very similar, ranging in size from 12.1 Mb in C. auris B11220 to 13.3 Mb in C. haemulonii , similar to that of C. lusitaniae (12.1 Mb) and other Candida species (Supplementary Table 2 ). Table 1 Genome assembly statistics of Candida auris and closely related species Full size table The assemblies of the C. auris clades are highly identical, sharing an average pairwise nucleotide identity of 98.7% across all four clades (I, II, III, and IV); clades II and III appear the most similar and share 99.3% identity. By contrast, comparison of nucleotide genome identity between species highlights greater interspecies genetic divergence: 88% between C. auris and each of the three related species ( C. haemulonii , C. duobushaemulonii , and C. pseudohaemulonii ), 89% between C. haemulonii and C. duobushaemulonii , and 92% between C. duobushaemulonii and C. pseudohaemulonii . To provide a quantitative measure of the degree of genetic variation within the C. auris population, we calculated the genome-wide nucleotide diversity ( π ) using SNPs identified from the isolate sequences of Lockhart et al. [2] . The estimated π is lowest for C. auris clade I (0.00050), and slightly higher for clades III and IV (0.00079 and 0.00075, respectively); π for all C. auris isolates is 0.0039, ~17-fold higher than the intra-clade levels. Comparing to other human fungal pathogens, this level of diversity is lower than that reported in Cryptococcus neoformans var. grubii , ( π = 0.0074 [20] ), but higher than the extreme clonality reported for Trichophyton rubrum ( π = 0.00054 [21] ). These comparisons support that the different clades of C. auris comprise a single species well separated from the related MDR species. As an independent assessment of the genome assembly size and structure, we generated optical maps of the C. auris B8441 and B11221 isolates (Supplementary Figure 1 ). Consistent with the assemblies of these isolates, the maps had seven linkage groups; nearly all of the genome assemblies were anchored to the optical maps (98.8% of B8441 and 97.2% of B11221; Supplementary Figure 1 ; Table 1 ). This supports the presence of seven chromosomes in C. auris , consistent with the chromosome number found in previous studies using electrophoretic karyotyping by pulsed-field gel electrophoresis (PFGE) [22] . While the genomes of C. auris are highly syntenic, we found evidence of a few large chromosomal rearrangements between C. auris B8441 and B11221 based on comparison of the assemblies and the optical maps (Fig. 1 , Supplementary Figure 1 ). We confirmed that the junctions of these rearrangements are well supported in each assembly; these regions show no variation in the depth of PacBio and Illumina aligned reads and there is no evidence of assembly errors across these rearrangement breakpoints. We additionally independently identified structural variants based on the read alignments to the B8441 and B11221 assemblies and recovered each of the rearrangements present in these assemblies. These large chromosomal rearrangements included one inversion of 136 kb between B8441 sc01 and B11221 sc01, a 274 kb translocation between B8441 sc08 and B11221 sc03, and a 300 kb translocation between B8441 sc10 and B11221 sc01 (Fig. 1 ). The genomes of C. auris , C. haemulonii , C. duobushaemulonii , and C. pseudohaemulonii showed limited chromosomal rearrangements between each other, mostly intra-chromosomal inversions between C. auris and C. haemulonii, C. duobushaemulonii , and C. pseudohaemulonii , and large chromosomal translocations between C. haemulonii , C. duobushaemulonii , and C. pseudohaemulonii (Fig. 1a ). These rearrangements between C. auris clades, and between species, could potentially prevent genetic exchange between these groups, since some crossover events will generate missing chromosomal regions or other aneuploidies and may result in nonviable progeny. Fig. 1 Whole genome conservation, structure, and synteny. a Genome wide gene synteny among Candida auris , C. haemulonii , C. duobushaemulonii , and C. pseudohaemulonii . To determine synteny regions of conserved gene order, we identified orthologs between these isolates and then plotted chains of orthologs (gray lines). Isolate names are shown to the left of their genomes, which are represented by horizontal black lines, with vertical lines indicating scaffold borders, and their identifiers listed above (+/− = orientation). b Shared synteny regions based on whole genome alignments between C. auris B8441 and B11221. Asterisk refers to scaffolds in reverse orientation Full size image Evolution of mating-type locus in C. auris and closely related species We characterized the mating type locus in C. auris and identified representatives of both mating types. The mating locus structure is highly conserved compared to closely related species including C. lusitaniae and other Saccharomycetales yeasts from the CTG clade Candida (Fig. 2 ). Many Candida species, including diploid asexual species, have heterothallic MTL idiomorphs, and mating occurs between cells of opposite mating type, MTL a and MTL α [23] . We found that the genes flanking the MTL locus in some species from the CTG clade Candida , namely the phosphatidylinositol kinase gene ( PIK1 ), the oxysterol binding protein gene ( OBP1 ), and the poly(A) polymerase gene ( PAP1 ), were adjacent in all sequenced genomes of the emerging MDR clade (Fig. 2a ). Previous work reported that the genome of C. auris 6684 included the MTL flanking genes but did not identify either MTL a or MTL α genes at this locus [13] . In the chromosome level genome assemblies of C. auris (B8441 and B11221), the PIK1/OBP1/PAP1 genes are present at a single locus in chromosome 3 in B8441 (sc05) and B11221 (sc03). Notably, we found all C. auris isolates contained either the MTL a and MTL α idiomorphs at this locus and that gene order was conserved compared to the C. lusitaniae MTL [24] (Fig. 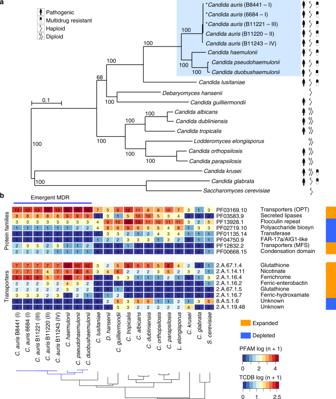Fig. 3 Phylogenomic and gene family changes inCandida aurisand related species.aMaximum likelihood phylogeny using 1570 core genes based on 1000 replicates, among 20 annotated genome assemblies, includingCandida auris, C. haemulonii(B11899),C. duobushaemulonii(B09383), andC. pseudohaemulonii(B12108), and closely related species. Branch lengths indicate the mean number of changes per site.bHeatmap depicting results of protein family enrichment analysis (PFAM domains; correctedp-value < 0.05) comparing the gene content ofC. aurisstrains representing each clade,C. haemulonii,C. duobushaemulonii, andC. pseudohaemulonii, and other closely related species, includingC. lusitaniae,C. albicans,C. krusei, andC. glabrata. Values are colored along a blue (low counts) to red (high counts) color scale, with color scaling relative to the low and high values of each row. Each protein family domain has a color code (right) indicating whether expanded or depleted 2a ; Supplementary Table 3 ). We found that the MTL a is present in C. auris B8441 and 6684 (clade I), B11243 (clade IV), and C. pseudohaemulonii , spanning 14.9 kb (Fig. 2a ). By contrast, C. auris B11220 (clade II), B11221 (clade III), and C. haemulonii and C. duobushaemulonii contain MTLα , spanning 14.3 kb (Fig. 2a ). Phylogenetic analysis of the non-mating flanking genes ( PIK1/OBP1/PAP1 ) supports the inheritance of idiomorphs of these genes with the MTL a and MTL α genes (Fig. 2b ). Upon further examination and manual annotation, we determined that a 1/ a 2 are present in MTL a isolates, and α1 is present in MTL α isolates; as in C. lusitaniae , the MTL α locus is missing the α2 gene [24] (Fig. 2a ). RNA-Seq data was used to guide gene prediction of a 1 and a 2, and further established that both genes are expressed in B8441 (Supplementary Figure 2 ), supporting the hypothesis that these genes could be functional, and that the MTL locus could be used to classify C. auris isolates. To further characterize the evolution of mating type in the population, we examined the MTL locus using 50 isolates from Lockhart et al. [2] and found that all isolates from clade I and IV have MTL a , whereas all isolates from clade II and III had MTL α (Fig. 2c , Supplementary Figure 3 ). The fact both a and α MTL alleles are present and expressed in C. auris suggests this species may be capable of mating, either in the ancestral population of the outbreak clades or if the expanding outbreak results in the presence of isolates from both mating types in a geographic area. Fig. 2 Mating-type loci ( MTL ) in Candida auris and closely related species. a Synteny schema depicting the orientation and conservation of the color-coded MTL idiomorphs and genes adjacent to the MTL . The putative MTL in C. auris , C. haemulonii , C. duobushaemulonii , and C. pseudohaemulonii are shown in comparison with the MTL a and MTL α idiomorphs from C. lusitaniae . b Phylogenetic analysis of the non-mating flanking genes ( PIK1/OBP1/PAP1 ) showing the inheritance of idiomorphs of these genes within the MTL a and MTL α loci. Branch lengths indicate the mean number of changes per site. c Phylogenetic tree of C. auris isolates from Lockhart et al. [2] . Isolates are color-coded according to the clades (I, II, III, and IV) and mating type ( MTL a and MTL α). Supplementary Figure 3 shows isolates, origin, and the normalized depth read coverage of mapped positions for all isolates aligned to B8441 ( MTL a ) and B11221 ( MTL α), supporting the classification into MTL a or MTL α Full size image We examined the conservation of genes involved in meiosis to provide additional support for potential mating in C. auris . We found that many of the key meiotic genes are similarly conserved between C. lusitaniae , Candida guilliermondii , C. auris , C. haemulonii , C. duobushaemulonii , and C. pseudohaemulonii (Supplementary Data 1 ). Some genes involved in meiosis in Saccharomyces cerevisiae appeared absent in these species including the recombinase DMC1 and cofactors ( MEI5 and SAE3 ), synaptonemal-complex proteins ( ZIP1 and HOP1 ), and genes involved in crossover interference ( MSH4 and MSH5 ; Supplementary Data 1 ). A small number of genes involved in meiosis were present in C. lusitaniae but absent in C. auris , C. haemulonii , C. duobushaemulonii , and C. pseudohaemulonii . In C. auris , the DNA recombination and repair genes RAD55 and RAD57 appear to be absent, however RAD55 is widely absent in the CTG Candida clade while the RAD51 paralog of the RAD55 / RAD57 complex is present. C. lusitaniae , despite the loss of many of the same meiotic genes, undergoes meiosis during sexual reproduction involving diploid intermediates [24] . The fact that most components of the mating and meiosis pathways are similarly conserved in C. auris and closely related species including C. lusitaniae suggest these species may have the ability to mate and undergo meiosis as observed for C. lusitaniae . Phylogenetic position of C. auris and closely related species Using the complete genomes, we estimated a strongly supported phylogeny of C. auris , C. haemulonii , C. duobushaemulonii , and C. pseudohaemulonii , relative to other species from the order Saccharomycetales including C. lusitaniae , C. tropicalis , C. albicans , and C. glabrata (Supplementary Table 2 ). Based on a concatenated alignment of 1570 single copy core genes, a well supported maximum likelihood tree placed C. auris , C. haemulonii , C. duobushaemulonii , and C. pseudohaemulonii as a single clade, confirming the close relationship of these species (100% of bootstrap replicates; Fig. 3a ). The C. auris clades appear more recently diverged based on short branch lengths within this species. Previous phylogenetic analyses had shown conflicting relationships between C. auris , C. haemulonii , C. duobushaemulonii , and C. pseudohaemulonii [4] , [5] , [12] , [13] . Our phylogenetic analysis strongly supports that C. duobushaemulonii and C. pseudohaemulonii are most closely related to each other, and form a sister group to C. haemulonii , which appeared as the more basally branching species (Fig. 3a ). The most closely related species to this MDR clade is C. lusitaniae , which is the more basally branching member of this group (Fig. 3a ). Fig. 3 Phylogenomic and gene family changes in Candida auris and related species. a Maximum likelihood phylogeny using 1570 core genes based on 1000 replicates, among 20 annotated genome assemblies, including Candida auris, C. haemulonii (B11899), C. duobushaemulonii (B09383), and C. pseudohaemulonii (B12108), and closely related species. Branch lengths indicate the mean number of changes per site. b Heatmap depicting results of protein family enrichment analysis (PFAM domains; corrected p -value < 0.05) comparing the gene content of C. auris strains representing each clade, C. haemulonii , C. duobushaemulonii , and C. pseudohaemulonii , and other closely related species, including C. lusitaniae , C. albicans , C. krusei , and C. glabrata . Values are colored along a blue (low counts) to red (high counts) color scale, with color scaling relative to the low and high values of each row. Each protein family domain has a color code (right) indicating whether expanded or depleted Full size image Gene family expansions linked to drug resistance and virulence Gene annotation of the C. auris genomes was performed using RNA-Seq paired-end reads to improve gene structure predictions (Methods). The predicted gene number was highly similar across all C. auris genomes as well as in C. haemulonii , C. duobushaemulonii , and C. pseudohaemulonii . In C. auris , the number of protein-coding genes varied between 5421 in B8441 and 5601 in B11243. 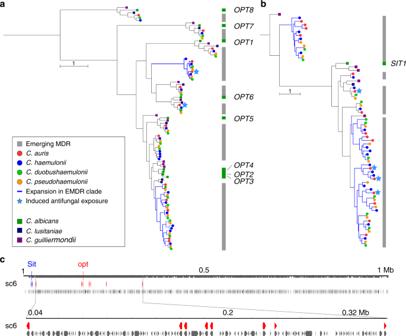Fig. 4 Phylogenetic relationships of expanded families of transporters.a,bMaximum likelihood phylogenetic trees showing expansion of oligopeptide transporters (OPT) and siderophore iron transporters (SIT) families inC. aurisandC. haemulonii,C. duobushaemuloniiandC. pseudohaemulonii. Each species has a color code and lineage-specific expansions (blue branches) can be seen inC. aurisand closely related species relative to the close ancestorC. lusitaniaeandC. albicans. Orthologs ofOPTandSITtransporters inC. albicansare depicted alongside each tree.cChromosome view depicting genes and orientation located in chromosome 6 (B8441 scaffold05). This region highlights expansion and tandem duplication of eightOPTclass transporters (in red) For C. haemulonii , C. duobushaemulonii , and C. pseudohaemulonii the numbers were very similar, ranging from 5288 to 5410 predicted genes (Table 1 ; Supplementary Figure 4a ). High representation of core eukaryotic genes provides evidence that these genomes are nearly complete; 96–98% of these conserved genes are found in all annotated genome assemblies (Supplementary Figure 1b ). By examining orthologous genes in C. auris , C. haemulonii , C. duobushaemulonii, C. pseudohaemulonii , and 12 additional Saccharomycetales genomes, including C. lusitaniae , C. tropicalis , C. albicans , and C. glabrata , we found a total of 2379 core ortholog clusters had representative genes from all 20 analyzed genomes (Supplementary Figure 4 ). We found a small number of unique genes in the C. auris clades ranging from 15 (B8441; clade I) to 54 (B11221; clade III) genes, and higher numbers in the three related species (203 in C. haemulonii , 83 in C. duobushaemulonii , and 88 in C. pseudohaemulonii ; Supplementary Figure 5 ). The unique genes in C. auris clades include oligopeptide and ABC transporters (Supplementary Data 2 ). While unique glycophosphatidylinositol (GPI)-anchored proteins were identified in C. auris , we found high conservation across C. auris , C. haemulonii , C. duobushaemulonii, C. pseudohaemulonii of seven (GPI)-anchored proteins ( PLB3 , IFF4 , PGA52 , PGA26 , CSA1 , HYR3 , and PGA7 ) that were upregulated during C. auris biofilm formation and are associated with antifungal resistance and biofilm mechanisms in C. albicans [25] (Supplementary Data 2 ). To characterize changes in gene content that differentiate C. auris , C. haemulonii , C. duobushaemulonii , and C. pseudohaemulonii from related species, we searched for expansions or contractions in functionally classified gene sets (Supplementary Table 2 ). We identified PFAM domains that were significantly enriched or depleted (Methods; Fig. 3b , Supplementary Figure 4 ). Domains associated with transmembrane transporters (OPT, MFS) and secreted lipases (LIP) were enriched in C. auris , C. haemulonii , C. duobushaemulonii , and C. pseudohaemulonii compared to other genomes ( q- value < 0.05, Fisher’s exact test; Fig. 3b ). We therefore further classified transmembrane transporters using the Transporter Classification Database (TCDB) and found that the higher copy number of transporters in the emergent MDR clade could be attributed to oligopeptide transporters ( OPT ) and siderophore iron transporters ( SIT ). In C. albicans , OPT transporters enable uptake of small peptides; the expression of some OPT transporters are up-regulated by azole drugs [26] , [27] . While most of the 14 OPT genes found in C. auris had orthologs in C. albicans ( OPT1–8 ), a subset of these transporters appear recently duplicated in the MDR emergent clade, including an expansion of three OPT1 -like transporters, and five transporters similar to OPT2 , OPT3 , and OPT4 (Fig. 4a , Supplementary Figure 6 ). Most of the OPT genes (up to 8) are located in a conserved locus among emerging MDR species encompassing 296 kb of chromosome 6; this gene family appears to have expanded by tandem duplication (Fig. 4c ). In C. albicans , iron transporters include the siderophore transporter SIT1 and the iron permeases FTR1 and FTR2 ; a subset of these transporters is uniquely expanded in C. auris and closely related species, including the expansion of 14 ortholog groups in C. auris related to C. albicans SIT1 (Fig. 4b , Supplementary Figure 6 ). Secreted lipases are also expanded in the genomes of C. auris and closely related species ( q- value < 0.05, Fisher’s exact test; Fig. 3b ). The C. auris clade has similar counts of lipases relative to C. albicans and Candida dubliniensis , however, these proteins are expanded relative to more closely related human pathogenic species, including C. lusitaniae , C. guilliermondii , Candida krusei , and C. glabrata (Fig. 3b ). Phylogenetic analysis suggested independent evolutionary trajectories of secreted lipases in emerging C. auris and related species, where the most recent ortholog family of lipases includes C. albicans LIP4 , 5 , 8 , and 9 (Supplementary Figure 7 ). The secretion of lipases may be important during infection for nutrient acquisition, adaptation, virulence, and immune evasion [28] ; we identified a predicted secretion signal in all lipases encoded by C. auris and related species, supporting an extracellular role in these emergent MDR species. Fig. 4 Phylogenetic relationships of expanded families of transporters. a , b Maximum likelihood phylogenetic trees showing expansion of oligopeptide transporters ( OPT ) and siderophore iron transporters ( SIT ) families in C. auris and C. haemulonii , C. duobushaemulonii and C. pseudohaemulonii . Each species has a color code and lineage-specific expansions (blue branches) can be seen in C. auris and closely related species relative to the close ancestor C. lusitaniae and C. albicans . Orthologs of OPT and SIT transporters in C. albicans are depicted alongside each tree. c Chromosome view depicting genes and orientation located in chromosome 6 (B8441 scaffold05). This region highlights expansion and tandem duplication of eight OPT class transporters (in red) Full size image Conservation of known drug resistance and virulence related genes The isolates selected for genome sequencing display increased resistance to antifungal drugs. Increased resistance to fluconazole is most commonly observed in C. auris with some isolates also displaying increased resistance to voriconazole or amphotericin B (Supplementary Table 1 [2] ). The three related species all displayed increased amphotericin B resistance, and two were also resistant to fluconazole. All isolates appeared sensitive to the echinocandins tested, anidulafungin and caspofungin (Supplementary Table 1 ). Most of the genes associated with drug resistance and pathogenesis in C. albicans are conserved in C. auris , C. haemulonii , C. duobushaemulonii , and C. pseudohaemulonii . We identified orthologs of genes noted to confer drug resistance in C. albicans , either by acquiring point mutations, increasing transcription, or copy number variation (CNV). The annotated genome assemblies of C. auris , C. haemulonii , C. duobushaemulonii , and C. pseudohaemulonii contain a single copy of the ERG11 azole target and the UPC2 transcription factor that regulates the expression of genes in the ergosterol pathway, as well as all the gene components of the ergosterol biosynthesis pathway (Supplementary Data 3 ). Several of the sites in ERG11 subject to drug-resistant mutations in C. albicans are similarly mutated in drug-resistant C. auris isolates (at positions Y132, K143, and F126, as reported previously [2] ). Analysis of the annotated genome assemblies of C. auris isolates agrees with prior SNP analysis [2] , with the exception of F126L mutation in B11221 (clade III), initially reported as F126T for this isolate though this was recently corrected to F126L [29] . The F126L mutation is also observed in a separate genomic study of C. auris [7] and in drug-resistant C. albicans [30] (Supplementary Figure 8 ). The Y132F mutation observed in two C. auris clades is also found in C. pseudohaemulonii , suggesting this site may contribute to the increased azole resistance of this C. pseudohaemulonii isolate (Supplementary Table 1 ). Other sites in ERG11 that confer drug resistance in C. albicans do not display drug-resistant mutations in C. auris , C. haemulonii , C. duobushaemulonii , and C. pseudohaemulonii (Supplementary Figure 8 ). In addition, we found that not all C. auris isolates have a single copy of ERG11 . Using CNV analysis of the Illumina read depth of 47 previously sequenced isolates, we found a total of 6 large duplicated regions (CNVnator p -value < 0.01) ranging in size from 12 to 153 kb (Supplementary Data 4 ; Methods). The largest duplicated region of 153 kb is present in two isolates (B11227 and B11229) from clade III and encompassed 62 genes including ERG11 (Supplementary Figure 9 ; Supplementary Data 4 ). These two isolates also display increased resistance to fluconazole (Supplementary Table 1 ). Long read assemblies of these isolates could be used to examine the chromosomal context of this duplication. Additionally, we identified orthologs of transporters from the ATP binding cassette ( ABC ) and major facilitator superfamily ( MFS ) classes of efflux proteins that are involved in clinical antifungal resistance in C. albicans by the overexpression of ABC transporter family CDRs ( CDR1 and CDR2 ) and the MFS transporter MDR1 [31] , [32] . We identified a single copy of the multidrug efflux pump MDR1 in all sequenced isolates (Table 2 ). We further characterized the presence of CDR genes and MDR1 in the C. auris population by examining CNV and gene conservation across the 47 isolates from Lockhart et al. [2] , and did not detect any CNV of these transporters across this set (Supplementary Data 5 ). Candidate multidrug transporters similar to CDR1 , CDR2 , and related genes include 5 genes in most genomes ( C. auris B8441, B11220, and B11243, C. haemulonii , and C. pseudohaemulonii ), 6 genes in C. auris B11221, and 4 genes in C. duobushaemulonii (Table 2 ; Supplementary Figure 10 ). Phylogenetic analysis of these ABC transporters showed that one of the genes in C. auris is related to CDR1 / CDR2 / CDR11 , two genes are related to CDR4 , and two genes are related to SNQ2 ; C. auris B11221 has an additional copy of SNQ2 (Supplementary Figure 10 ). The TAC1 transcription factor that regulates the expression of CDR1 and CDR2 in C. albicans is present in two tandem copies in C. auris , C. haemulonii , C. duobushaemulonii , and C. pseudohaemulonii (Table 2 ). Table 2 Conservation of genes involved in pathogenesis and drug resistance Full size table While many gene families involved in pathogenesis in C. albicans are present in similar numbers in C. auris , C. haemulonii , C. duobushaemulonii , and C. pseudohaemulonii , there are some notable differences such as of cell wall and transmembrane proteins. We identified similar numbers of the secreted aspartyl proteases, lipases and oligopeptide transporters ( OPT ), and only one copy of the ALS cell surface family of C. albicans (Table 2 ). We also examined whether other genes involved in the C. albicans core filamentation response were conserved in the emerging MDR species (Supplementary Data 2 ). While most of these genes are conserved in C. auris and closely related species, two genes are absent, candidalysin ( ECE1 ) and the hyphal cell wall protein ( HWP1 ), both of which are highly expressed in C. albicans hyphae [33] , [34] . Thus, we additionally assessed if any other cell surface families of proteins are enriched in C. auris and closely related species. We found a total of 75 genes with a predicted GPI anchor, including genes that were found only in the emerging MDR clade, including one unique family expanded in C. auris (Supplementary Data 2 ). The most represented protein family domains in these genes included the N-terminal cell wall domain, the aspartyl protease domain, and the fungal-specific cysteine-rich (CFEM) domain (Supplementary Data 2 ). The shared profile of these genes across C. auris and other MDR species suggests that the more rarely observed species may be similarly primed to become more common human pathogens. Transcriptional C. auris response to voriconazole and amphotericin B To investigate which C. auris genes are involved in antifungal resistance, we carried out RNA-Seq of C. auris strains B8441 and B11210 (clade I) to profile gene expression changes after exposure to two antifungal drugs, voriconazole (VCZ) and amphotericin B (AMB). B11210 is resistant to AMB and exhibits an elevated MIC to VCZ, while B8441 is susceptible to AMB and displays a low MIC to VCZ (Supplementary Table 1 [2] ). We identified differentially expressed genes (DEGs) in B8441 and B11210 after 2 and 4 h of drug exposure (Methods; Supplementary Table 4 ; Supplementary Figure 11a ). The response of the susceptible  isolate B8441 to AMB or VCZ involved increased expression of small sets of genes: 39 genes were induced in response to AMB, 21 in response to VCZ, of which 14 were induced by both drugs (fold change (FC) > 2; false discovery rate (FDR) < 0.05; Supplementary Figure 11b ). Genes induced upon AMB exposure were enriched in small molecule biosynthetic process and iron homeostasis (enriched GO terms corrected- p < 0.05, hypergeometric distribution with Bonferroni correction; Supplementary Data 6 ). Notably, this set includes genes involved in the C. albicans transcriptional response to AMB associated with transport and with lipid, fatty acid, and sterol metabolism [35] including genes involved in arginine synthesis ( ARG1 / ARG3 ), ergosterol biosynthesis ( ERG24 ), fatty-acid metabolism ( FAS1 / FAS2 ), GPI-linked surface proteins ( PGA7 and RBT5 ), and several iron transporters (class FTH1 and SIT1 ; Supplementary Data 6 ; Figure S11c ). Three of these genes ( SIT1 , PGA7 , and RBT5 ) have also been found to be upregulated during C. auris biofilm formation [25] , suggesting that cell wall reorganization may be part of the drug response. Genes induced in B8441 in response to both AMB and VCZ were enriched in transmembrane transport and iron transport categories (enriched GO terms corrected- p < 0.05, hypergeometric distribution with Bonferroni correction), including a ferric reductase ( FRP1 ), a high affinity iron transporter ( FTH1 ), a glucose transporter ( HGT7 ), a N-acetylglucosamine transporter ( NGT1 ) and an oligopeptide transporter ( OPT1-like ; Supplementary Data 6 ). Genes only induced with VCZ included the oligopeptide transporter PTR22 . We also examined expression differences in the resistant isolate B11210. As a large set of genes was identified as differentially expressed compared to the control sample, we focused on the most highly induced or repressed genes (FC > 4; FDR < 0.001; Supplementary Figure 11a ). A total of 106 genes were induced in response to AMB and 41 genes in response to VCZ, of which 40 were commonly induced (Supplementary Figure 11b ). Genes induced in response to AMB were enriched in transcription and translation processes and in sterol biosynthetic process (enriched GO terms corrected- p < 0.05, hypergeometric distribution with Bonferroni correction). Notably, 5 of the 21 genes involved in the ergosterol biosynthesis pathway were highly induced in B11210, including MVD , ERG2 , ERG1 , ERG6 , and ERG13 (Supplementary Data 6 ; Supplementary Figure 11b ; Supplementary Figure 12 ). This correlates with the maintenance of cell membrane stability, as previously noted for the transcriptional response of C. albicans to AMB, since AMB binds to ergosterol in the cell membrane [35] . Genes induced by both drugs in B11210 are enriched in amide biosynthetic process and translation, and genes only induced by VCZ are enriched in RNA processing and transcription (enriched GO terms corrected- p < 0.05, hypergeometric distribution with Bonferroni correction; Supplementary Data 6 ). Since C. auris isolates B8441 and B11210 (clade I) had disparate resistance phenotypes predominantly in response to AMB, we further examined expression changes between these two strains. Despite the fact that B8441 and B11210 are from the same clade (clade I) only 8 genes were induced in both strains upon AMB treatment, including ARG1 , CSA1 , and MET15 , and one OPT1 -like transporter (B9J08_001998; Supplementary Data 7 ). In addition, comparison of both isolates before the treatment revealed that the resistant strain B11210 has higher expression of genes previously noted to be involved in the C. albicans transcriptional response to drug exposure relative to B8441 even in the absence of drug (Supplementary Data 8 ). This set of genes encompasses the D-xylulose reductase ( XYL2 ) [35] , phosphoenolpyruvate carboxykinase ( PCK1 ) [26] , [35] , and a large set of transporters ( FRP1 , FTH1 , HGT13 , HGT7 , HSP70 , NGT1 , OPT1 , PTR22 , SEC26 ) [35] , which suggests intrinsic expression of genes associated with polyene resistance in B11210 (Supplementary Data 7 ). In addition, we observed that the expression levels of homologs of multidrug transporters ( CDR1 , CDR4a , CDR4b , MDR1 , SNQ2 ) did not significantly vary across exposure to either drug or between isolates. Of these, CDR4a appears more highly transcribed relative to other multidrug transporters ( CDR1 , MDR1 , or SNQ2 ). This supports previous findings of intrinsic higher expression of transporters as a possible mechanism of drug resistance in C. auris [12] . We compared these results to SNP variants identified between B8441 and B11210 to evaluate if any may explain the phenotypic difference in drug resistance in these strains. We found a total of 1148 SNPs and 430 insertion or deletion events (Supplementary Data 8 ). A total of 15 genes display a loss of function mutation (frame-shift, stop gained or stop lost), including the stationary phase protein (SNZ1) and the putative GPI-anchored adhesin-like protein ( HYR3 ). We did not find loss of function mutations in genes previously associated with amphotericin B resistance in C. albicans , however, we did identify non-synonymous mutations in genes associated with drug resistance and response to amphotericin B, including ERG11 , ERG4 , CDR1 , C5_05230C_A , NHP6A and other transporters such as HGT7 and YCF1 (Supplementary Data 8 ). These variants suggest candidate mutations that could explain phenotypic variation in drug resistance, however a wider association study of mutations and drug resistance levels would help identify the major genes involved across the different clades. While many genes associated with antifungal resistance are conserved across C. auris and CTG species, unique genes and gene duplication in C. auris may also contribute to the underlying emergence of MDR phenotypes. Some genes induced by AMB or VCZ in C. auris B8441 and B11210 (Supplementary Data 7 ) were specific to C. auris or to the emerging clade of C. auris , C. haemulonii , C. duobushaemulonii , and C. pseudohaemulonii . This includes five ortholog families unique to C. auris , comprising three putative GPI-anchored cell wall proteins, two homologs of IFF6 (a putative GPI-anchored adhesin-like protein), one homolog of PGA54 , and an aspartyl protease similar to SAP8 (Supplementary Data 6 ). In addition, this set included gene families that are expanded in C. auris or in closely related species (Figs. 3b and 4 ), including transporters (four SIT -like, one FTR -like, and two OPT -like class), cell wall adhesins, and several predicted secreted proteins (Supplementary Data 6 ). Notably, while other Saccharomycetales species including C. albicans only have one copy of SIT1 that is induced during AMB treatment, C. auris and closely related species had up to 11 SIT1 -like genes, of which 4 are induced during AMB treatment (Fig. 3b , Supplementary Figure 6 ). Together, these transcriptional changes highlighted shared and C. auris -specific genes that might contribute to the MDR phenotype observed in C. auris isolates and provided candidate genes to further investigate C. auris multidrug-resistance. As an emerging pathogen, C. auris has not been well studied to date, highlighting the need for rapidly closing this knowledge gap to respond to the increasing number of fatal infections. There is also a limitation on how much of the biology of C. auris we can infer from related Candida species; C. auris is distantly related to the two most commonly observed pathogenic Candida species, C. albicans and C. glabrata , as well as other sequenced species. Our comparative genomic analyses, incorporating new genomic data for more closely related, MDR species, revealed the recent evolution of this group of emerging pathogens including shared properties that underlie antifungal resistance and virulence. In addition to C. auris clades, we generated annotated genomes for three other closely related species rarely observed as infecting humans. Building on prior studies of individual loci [4] , [5] , [12] , [13] , the phylogenetic relationship of these species was more clearly resolved by whole genome comparisons; C. haemulonii , C . duobushaemulonii , and C. pseudohaemulonii are more closely related to each other than to C. auris , with the closest relationship being between C . duobushaemulonii and C. pseudohaemulonii . Our phylogenetic analysis integrating the genomes of these species with other Candida highlights the distant relationship of this group to other pathogenic Candida species and the placement of these species within the CTG clade. To characterize mechanisms that may contribute to virulence and drug resistance, we compared the gene content between the emerging MDR species and other related Candida . Recent work found that virulence in C. auris appears similar to C . albicans and C . glabrata [36] , suggesting that shared gene content could play a role. C. auris shares some notable gene family expansions described in C. albicans and related pathogens [23] , including of transporters and secreted lipases. While an expansion of transporters is shared, species-specific expansions have contributed to the diversification of transporters in C. auris and closely related species. Similarly, the expansion of lipases suggests this could be part of a shared mechanism of virulence; however, the roles of specific genes will need to be investigated. In contrast, expansions of cell wall families detected in C. albicans and related pathogens are not found in C. auris and related species. For example, the ALS family is represented by two to four copies in C. auris and related MDR species, compared to the eight copies present in C. albicans . Examining the predicted cell wall proteins in C. auris did not reveal any highly expanded families; perhaps the longer history of association with humans has impacted diversification of such cell wall protein families in the more commonly observed pathogenic Candida species. Drug resistance in C. auris likely involves mechanisms previously described in C. albicans , however the specific transporters involved in drug response are less conserved. All four species are resistant to antifungal drugs, and the Y132F mutation in the azole drug target ERG11 , previously described in C. auris , and was also detected in C. pseudohaemulonii . The direct link between these mutations and azole resistance in C. auris is supported by a recent work that found that expression of either the Y132F and K143R C. auris ERG11 allele led to an increase in azole resistance in a heterologous system [17] . In addition, we find evidence of increased copy number of ERG11 in two C. auris isolates, but little evidence of multiple isolates with regions of CNV, and no evidence of aneuploidy. This suggests that increased copy number of ERG11 may be a mechanism of drug resistance in C. auris , as has been described in C. albicans [37] . However other mechanisms of drug resistance may vary between species and strains. For example, we found that efflux proteins such as the CDR family were not induced during voriconazole treatment, instead other transporters were up-regulated, including those that are either expanded or unique in C. auris and closely multidrug emergent species, highlighting that different molecular mechanisms are likely involved in the drug response. Our analysis identified representative C. auris isolates for each of the two mating types, suggesting that this species has the potential to undergo mating and meiosis. Each of the four described C. auris clades consists of isolates that are all MTL a or MTL α; as the clades are geographically restricted, this suggests that there is a geographic barrier to opposite-sex mating. This expectation would change if wider sampling demonstrated the establishment of both mating types within a geographic area. The potential for mating within this species is supported by the conservation of genes involved in mating and meiosis; these patterns are similar to that of the related species C. lusitaniae , for which mating and recombination have been demonstrated [24] . Isolates from clades of opposite mating types could be directly tested for mating and production of progeny. One potential barrier to mating between clades is the presence of chromosomal rearrangements, as some recombination events may result in inviable progeny. Analyses of these genomes have revealed fundamental aspects of these emerging MDR fungi. The role of specific genes in mating, drug resistance, or pathogenesis needs to be directly tested, utilizing gene deletion technologies recently adapted for C. auris (e.g., ref. [38] ). Further analysis of this data will not only advance our understanding of the basis of drug resistance and virulence of this pathogen but can also inform the development of fungal diagnostics for accurate tracking of these emerging pathogens. Selected isolates and genome sequencing Details of the strains used in this study are presented in Table 1 and additional details were previously reported [2] , [18] , [19] . Isolates were grown on Sabouard Dextrose media supplemented with chloramphenicol and gentamycin and incubated for 24–48 h at 37 °C. For Illumina sequencing, genomic DNA was extracted using the Quick -DNA™ (ZR) Fungal/Bacterial Miniprep Kit (Zymo Research, Irvine, CA, USA). Genomic libraries were constructed and barcoded using the NEBNext Ultra DNA Library Prep kit (New England Biolabs, Ipswich, MA, USA) by following manufacturer’s instructions. Genomic libraries were sequenced using either Illumina HiSeq 2500 with HiSeq Rapid SBS Kit v2 or Illumina MiSeq platform using MiSeq Reagent Kit v2 (Illumina, San Diego, CA, USA). For PacBio sequencing, DNA was extracted using MasterPure™ Yeast DNA Purification Kit (Epicenter, Madison, WI, USA). Single-molecule real-time (SMRT) sequencing was done using the PacBio RS II SMRT DNA sequencing system (Pacific Biosciences, Menlo Park, CA, USA). Specifically, 20-kb libraries were generated with the SMRTbell Template Prep Kit 1.0 (Pacific Biosciences). Libraries were bound to polymerase using the DNA/Polymerase Binding Kit P6v2 (Pacific Biosciences), loaded on two SMRTcells (Pacific Biosciences), and sequenced with C4v2 chemistry (Pacific Biosciences) for 360 min movies. Genome assemblies The genomes of B8441 and B11221 C. auris isolates were assembled using the SmrtAnalysis suite v2.3 (Pacific Biosciences) [2] , [39] . C . haemulonii and C . duobushaemulonii genomes were assembled using Canu v1.6 [40] . The resultant contigs were checked for further joins and circularity using Circlator v1.5 [41] . The final contigs were polished using Quiver, part of SmrtAnalysis suite v2.3 (Pacific Biosciences) [39] . The sequence order for the chromosomes was verified using restriction enzyme AflII Whole Genome Mapping (OpGen, Gaithersburg, MA). The sequenced Illumina reads of C. auris (B11220 and B11243), and C. pseudohaemulonii (strain B12108) were assembled using the SPAdes assembler v3.1.1 [42] . Next, Pilon v1.16 [43] was used to polish the best assembly of each isolate, resolving single nucleotide errors (SNPs), artifactual indels, and local mis-assemblies. All genome assemblies were evaluated using the GAEMR package ( http://software.broadinstitute.org/software/gaemr/ ), which revealed no aberrant regions of coverage, GC content or contigs with sequence similarity suggestive of contamination. Scaffolds representing the mitochondrial genome were separated out from the nuclear assembly. All genome assemblies have been deposited at deposited at DDBJ/EMBL/GenBank (see Data availability statement). To address if any strain representing each C. auris clade could be uniformly diploid, we examined candidate heterozygous positions predicted by Pilon v1.12 [43] using mapped Illumina data. The low frequency and the absence of such positions supported that all sequenced genomes are homozygous haploids. Optical mapping Two strains of C. auris (B11221 and B8441) were compared by the OpGen optical mapping platform (OpGen, Inc., Gaithersburg, MD). High molecular weight genomic DNA from overnight grown cells were purified with Argus HMW DNA Isolation Kit (OpGen, Inc.) and examined for quality and concentration using the ARGUS QCards (OpGen, Inc.). The software program Enzyme Chooser (OpGen, Inc.) identified BamHI restriction endonuclease to be optimal for optical map production, because its cleavage of reference genomes would result in fragments that average 6–12 kbp in size, with no fragments larger than 80 kbp. Single genomic DNA fragments were loaded onto a glass surface of a MapCard (OpGen, Inc.) using the microfluidic device, washed and then digested with BamHI restriction enzyme, and stained with JOJO-1 dye through the ARGUS MapCard Processor (OpGen, Inc.). Map cards were scanned and analyzed by automated fluorescent microscopy using the ARGUS Whole Genome Mapper (OpGen, Inc.). The single molecule restriction map collections were then tiled according to overlapping fragment patterns to produce a consensus whole genome map. This map was imported into MapSolver (OpGen, Inc.) along with predicted in silico maps of contigs derived from WGS, using the same restriction enzyme for ordering and orientation of contigs during genome circularization. In-silico predicted optical maps of complete genomes were scaled according to the size of sequenced genomes to show identity with Optical maps (Supplementary Figure 1 ). RNA-Seq of B8441 and B11210 during drug treatment For RNA extraction, C. auris cells were grown in YPD broth medium (Difco Laboratories, Sparks, MD) at 30 °C in a shaking incubator at 300 rpm. After 18 h, the stationary phase cells were diluted with the equal volume of fresh YPD broth and incubated for 2 h at 37 °C to induce growth. After that, the cells were treated with amphotericin B at the final concentration of 0.25 µg/mL or voriconazole at the final concentration of 1 µg/mL (Sigma-Aldrich, St. Louis, MO) and incubated at 30 °C for additional 2 and 4 h in the presence of drug. Cells were centrifuged for 2 min at 12,000× g , pellets were flash frozen in dry ice/ethanol bath and stored at −80 °C. RNA was isolated using RiboPure™-Yeast rapid RNA isolation kit (Life Technologies, Carlsbad, CA) using the manufacturer’s protocol. RNA was adapted for sequencing using the RNAtag-Seq approach [44] , with the modification that the yeast RiboZero reagent was used for rRNA depletion. For each condition, two biological replicates were performed, and the read counts per transcript were highly correlated between replicates ( R > 0.90). Gene annotation Gene annotation in C. auris was performed using RNA-Seq paired-end reads to improve gene calling and structure predictions. Briefly, we mapped RNA-Seq reads to the genome assembly using Tophat2, and used the alignments to predict genes using BRAKER1 [45] , that combines GeneMark-ET [46] and AUGUSTUS [47] , incorporating RNA-Seq data into unsupervised training and subsequently generates ab initio gene predictions. Additionally, we re-annotated the genome of the 6684 strain [13] improving its gene set and predicted gene structures. tRNAs were predicted using tRNAscan [48] and rRNAs predicted using RNAmmer [49] . Genes containing PFAM domains found in repetitive elements or overlapping tRNA/rRNA features were removed. Genes were named and numbered sequentially. For the protein coding-gene name assignment we combined HMMER PFAM/TIGRFAM, Swiss-Prot, and KEGG products. For comparative analysis genes were functionally annotated by assigning PFAM domains, GO terms, and KEGG classification. HMMER3 [50] was used to identify PFAM domains using release 27. GO terms were assigned using Blast2GO [51] , with a minimum e -value of 1 × 10 −10 . Protein kinases were identified using Kinannote [52] and transporter families using TCDB version 01-05-2017 [53] . To evaluate the completeness of predicted gene sets, the representation of core eukaryotic genes was analyzed using CEGMA genes [54] and BUSCO [55] . Copy number variation and nucleotide diversity To identify regions in C. auris that exhibit CNV we analyzed Illumina read depth of 47 previously sequenced isolates. We identified genomic windows (1 kb) showing significant variation ( p -value < 0.01) in normalized read depth using CNVnator v0.3 [56] . To measure nucleotide diversity, we used SNPs identified from the isolate sequences of Lockhart et al. [2] . We computed genome-wide π using VCFtools v0.1.12 [57] for non-overlapping sliding windows of 5 kb for C. auris clade I, II, III, and all isolates. Comparative genomics and phylogenomic analysis To examine the phylogenetic relationship of the emerging MDR clade, including C. auris , C. haemulonii , C. duobushaemulonii , and C. pseudohaemulonii , we identified single copy orthologs in these sequenced genomes and 12 related species using OrthoMCL v1.4 [58] (Markov index 1.5; maximum e -value 1e−5). A total of 1570 protein-coding genes that have one single copy and are conserved in all 20 genomes were aligned using MUSCLE, and a phylogeny was estimated from the concatenated alignments using RAxML v7.7.8 [59] with model PROTCATWAG with a total of 1000 bootstrap replicates. To compare gene family expansion and contractions, we used orthologous gene clusters that we classified as core, auxiliary, and unique. We then searched for expansions or contractions in functionally classified genes by assigning PFAM domains, GO terms, and KEGG classification. Using a matrix of gene class counts for each classification type, we identified enrichment comparing the emerging MDR clade with all the other related species using Fisher’s exact test. Fisher’s exact test was used to detect enrichment of PFAM, KEGG, GO terms, and transporter families between groups of interest, and p -values were corrected for multiple comparisons [60] . Significant (corrected p -value < 0.05) gene class expansions or depletions were examined for different comparisons. Transcriptional analysis of C. auris RNA-Seq RNA-Seq reads were aligned to the transcript sequences of C. auris B8441 or B11221 using Bowtie2 [61] . Transcript abundance was estimated using RSEM (RNA-Seq by expectation maximization; v.1.2.21) as transcripts per million (TPM). TPM-normalized “transcripts per million transcripts” (TPM) for each transcript were calculated, and differentially expressed transcripts were identified using edgeR [62] , all as implemented in the Trinity package version 2.1.1 [63] . Genes were considered differentially expressed only if they had a 2-fold change difference (>2 FC) in TPM values and a FDR below or equal to 0.05 (FDR < 0.05), unless specified otherwise. To determine major patterns of antifungal-response specific we clustered gene expression patterns by k -means. To identify functional enrichment of DEGs, we used functional gene assignations from PFAM, GO terms, and KEGG (see Gene annotation), and then performed comparisons with Fisher’s exact test. To identify possible functions of the gene products of significantly differentially expressed drug resistance genes, protein homologs were assigned based on orthology, functional assignments (GO, PFAM, TIGRFAM), and experimental evidence from Candida genome database ( http://www.candidagenome.org ). Antifungal susceptibility testing Antifungal susceptibility testing was performed on isolates according to Clinical and Laboratory Standards Institute (CLSI) guidelines [64] . Custom prepared microdilution plates (Trek Diagnostics, Oakwood Village, OH, USA) were used for generating both azole and echinocandin susceptibilities while Etest® strips (BioMerieux, Marcy l’Etoile, France) were used for amphotericin B susceptibilities. Interpretive breakpoints for C. auris and related species do not exist but have been conservatively based on those breakpoints established for other Candida species.